COP1 E3 ligase protects HYL1 to retain microRNA biogenesis Constitutive photomorphogenic 1 (COP1) is a RING-finger E3 ligase that plays a central role in photomorphogenesis by destabilizing many light-regulated transcription factors and photoreceptors. Here, we reveal a novel function for COP1 E3 ligase in controlling global miRNA biogenesis in Arabidopsis thaliana . In cop1 mutants, the level of miRNAs is dramatically reduced because of the diminution of HYPONASTIC LEAVES 1 (HYL1), an RNA-binding protein required for precise miRNA processing. HYL1 is destabilized by an unidentified protease, which we tentatively call protease X, that specifically cleaves the N-terminal region from HYL1, thus neutralizing its function. Our results further show that the cytoplasmic partitioning of COP1 under light is essential to protect HYL1 against protease X. Taken together, we suggest a novel regulatory network involving HYL1, protease X, COP1 and light signalling that is indispensable for miRNA biogenesis in Arabidopsis thaliana . MicroRNAs (MiRNAs) are integral regulatory small RNA elements for many biological processes in eukaryotes. In animals, Drosha initiates processing of long primary transcripts into precursor miRNAs (pre-miRNAs) while Dicer generates miRNAs from pre-miRNAs [1] , [2] , [3] . In plants, the two-stepwise miRNA processing pathway requires three core proteins; Dicer-like protein 1 (DCL1) and two guiding proteins, HYPONASTIC LEAVES 1 (HYL1) and SERRATE (SE) [4] , [5] , [6] . In addition to the core processing proteins, at least 10 components have been reported that play direct or indirect roles in the intricate regulation of miRNA biogenesis [7] , [8] , [9] , [10] , [11] , [12] , [13] . To further isolate hidden components in miRNA biogenesis, we have developed a rapid and simple miRNA detection method using DNA-templated silver nanoclusters (DNA/AgNCs) probes [14] , [15] , [16] , [17] . By applying this method, we isolated COP1 E3 ubiquitin ligase that negatively regulates photomorphogenesis triggered by far-red and visible light. As a tagger for proteolysis, COP1 desensitizes many transcription factors and photoreceptors in the light signalling pathway of plants [18] , [19] , [20] . COP1 has roles in transcriptional, flowering, hormonal, circadian clock regulations and ultraviolet tolerances [21] , [22] . However, to date, neither the integration of COP1 nor of light signalling into miRNA biogenesis has been discussed. Moreover, the function of cytoplasmic COP1 in response to light has not yet been fully addressed, though its feature of shuttling between the nucleus and cytoplasm is important in the light-dependent developments. Through various approaches, we here show that HYL1, an essential factor for pri-miRNA processing, is rapidly degraded by an unknown protease and the proteolytic regulation is dynamically modulated by COP1 in response to light-to-dark transition, implying the integration of light signalling into miRNA biogenesis. COP1 deficiency compromises miRNA biogenesis The DNA/AgNCs probes encapsulate highly fluorescent AgNCs within an hour and the presence of target miRNA can be immediately monitored by the extinguishing of fluorescence ( Fig. 1a ). With the novel nanotech-based method, we found a significant reduction of miR166 and miR172 in cop1 . Unlike the notable drops of fluorescence when the DNA/AgNCs probes were mixed with the total RNA from wild type, the addition of total RNA from hyl1-2 and cop1-6 to the DNA/AgNCs probes showed much higher emission intensity than those of wild type ( Fig. 1b , Supplementary Fig. 1 ). The highest I 0 / I values (folds emission-drop) of two sensors seen for wild type were 12±2.3 (miR166) and 38±12 (miR172) fold, while the lower values seen for hyl1-2 were 2.1±0.4 and 3.4±1 and for cop1-6 were 4.5±2 and 3.8±1.1 ( Fig. 1c ). To confirm the reduction of miRNAs in cop1 , we performed conventional small RNA blot analyses and observed highly compromised levels of miRNAs in cop1-4 and cop1-6 ( Fig. 1d ). Encouraged by these results, using the Illumina platform, we generated 32, 32, 28 and 30 million clean reads that perfectly matched the Arabidopsis genome from the small RNA populations in cop1-4 , cop1-6 , hyl1-2 and wild type, respectively. We compared the normalized counts of mature miRNAs in cop1-4 , cop1-6 , hyl1-2 and wild type, and found that the majority of miRNAs were reduced in co p1-4 , cop1-6 and hyl1-2 ( Fig. 1e ). Out of the 84 miRNAs that had total expression of at least six transcripts per 10 million (TPTM), 78 (93%), 74 (88%) and 83 (99%) miRNAs showed reduced expression in cop1-4 , cop1-6 and hyl1-2 , respectively. Most of the miRNAs, whose expressions declined in cop1-4 (97%) and cop1-6 (86%), were reduced to 50% or lower as compared with the wild type ( Supplementary Data 1 ). The profiles of downregulated miRNAs mostly overlapped (82%) between hyl1-2 and the cop1 alleles ( Supplementary Fig. 2a ). The length distributions of trimmed reads also showed a similar pattern between hyl1-2 and cop1-4 , the distinctive reduction of 16–24 nt fragments and the subsequent increase of 30–40 nt fragments ( Supplementary Fig. 2b,c ). These results show that COP1, one of the well-characterized E3 ligases in eukaryotes, is extensively involved in miRNA biogenesis. 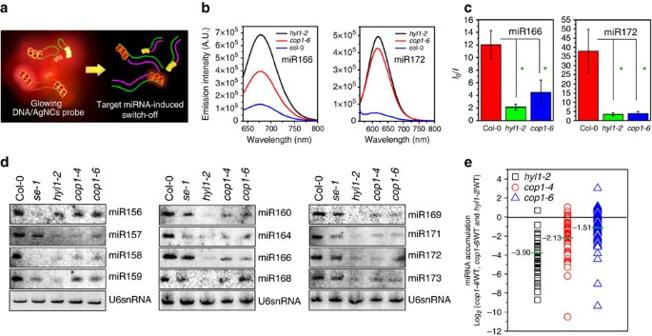Figure 1:COP1deficiency compromises miRNA biogenesis. (a) Schematic diagram for the DNA/AgNCs-probe based miRNA detection method. (b) Determination of the levels of miR166 and miR172 in WT,hyl1-2andcop1-6using the DNA/AgNCs probes. The fluorescent intensity is inversely correlated to the levels of target miRNA. The data were collected as the average value of three biological samples with ±s.d. (n=9). (c) Target sensibility of probes was shown inI0/Ivalues (I0andIare the emission intensity values without and with addition of total RNAs, respectively). TheI0/Iintensity versus total RNAs ofcop1-6,hyl1-2and wild type were given. The lower emission intensity represents the higher amount of target miRNA. The data were collected as the average value of three biological samples with ±s.d. (n=9). Significant differences between control and mutant alleles were indicated with asterisks (P<0.0001, student’st-test). (d) Small RNA blot analyses display the remarkably reduced miRNA levels incop1-4andcop1-6. U6snRNA used as loading control. (e) Illumina small RNA sequencing analysis confirmed the highly reduced miRNAs in mutant backgrounds. Figure 1: COP1 deficiency compromises miRNA biogenesis. ( a ) Schematic diagram for the DNA/AgNCs-probe based miRNA detection method. ( b ) Determination of the levels of miR166 and miR172 in WT, hyl1-2 and cop1-6 using the DNA/AgNCs probes. The fluorescent intensity is inversely correlated to the levels of target miRNA. The data were collected as the average value of three biological samples with ±s.d. ( n =9). ( c ) Target sensibility of probes was shown in I 0 / I values ( I 0 and I are the emission intensity values without and with addition of total RNAs, respectively). The I 0 / I intensity versus total RNAs of cop1-6 , hyl1-2 and wild type were given. The lower emission intensity represents the higher amount of target miRNA. The data were collected as the average value of three biological samples with ±s.d. ( n =9). Significant differences between control and mutant alleles were indicated with asterisks ( P <0.0001, student’s t -test). ( d ) Small RNA blot analyses display the remarkably reduced miRNA levels in cop1-4 and cop1-6 . U6snRNA used as loading control. ( e ) Illumina small RNA sequencing analysis confirmed the highly reduced miRNAs in mutant backgrounds. Full size image COP1 is an important element for the expression of HYL1 Subsequently, we investigated how COP1 integrates the regulatory layers of miRNA biogenesis. Since COP1 conjugates ubiquitin polymers to target proteins for their subsequent degradation by 26S proteasome, the target proteins of COP1 (for example, HFR1, LAF1, HY5 and PHYA) are in general accumulated in cop1 mutant lines [20] , [23] ( Supplementary Fig. 3c ). Thus, to understand the role of COP1 in miRNA biogenesis, we investigated the levels of major microprocessor components such as HYL1, SERRATE and DCL1 in cop1 using immunoblot analysis. In contrast to the accumulative pattern of the well-known targets, the level of HYL1 was significantly diminished in cop1-4 and cop1-6 , whereas DCL1 and SERRATE proteins were relatively unaffected ( Fig. 2a ). The reduced level of HYL1 coincided with the level of COP1 in cop1-4 and cop1-6 , showing a correlation between the two proteins ( Fig. 2a and Supplementary Fig. 3d ). Interestingly, we observed the immensely accumulated DCL1 levels in hyl1-2 and se-1 , as well as the increased level of SERRATE in hyl1-2 , implying that an unidentified feedback regulatory network may exist among those microprocessor components in which COP1 is not engaged ( Fig. 2a ). 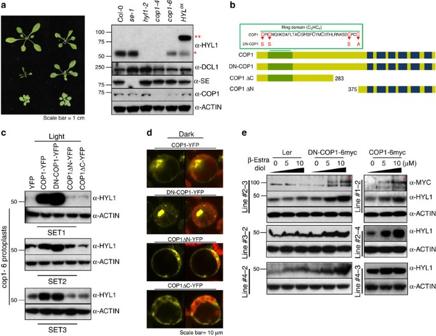Figure 2: COP1 is an important element for sustaining the expression of HYL1. (a) Immunoblot analysis shows that the level of HYL1 is highly diminished incop1-4andcop1-6. DCL1 is dramatically accumulated inhyl1-2andse-1. SERRATE and DCL1 are maintained incop1alleles. Single asterisk means endogenous HYL1; double asterisk means HYL1–6myc. Left panel displays the morphological characteristics of WT and mutants. (b) The cartoon shows the details of transient gene constructs. (c) Transient-complementation assays. Transiently expressed COP1-YFP and DN-COP1-YFP successfully restored the level of HYL1 incop1-6protoplasts in contrast to COP1ΔN-YFP, COP1ΔC-YFP and YFP that were unsuccessful. (d) The expression of transfected genes were determined by confocal microscopy. (e) The levels of HYL1 in WT/XVE-DN-COP1-6mycand WT/XVE-COP1-6myctransgenic plants, which have grown in β-estradiol supplemented medium for 10 days. The experiments were commenced with three individual transgenic lines. The levels of HYL1 were determined with α-HYL1 antibody. Induced DN-COP1 and COP1 were determined with α-Myc antibody. Equal loading of samples was determined with α-actin antibody. Figure 2: COP1 is an important element for sustaining the expression of HYL1. ( a ) Immunoblot analysis shows that the level of HYL1 is highly diminished in cop1-4 and cop1-6 . DCL1 is dramatically accumulated in hyl1-2 and se-1 . SERRATE and DCL1 are maintained in cop1 alleles. Single asterisk means endogenous HYL1; double asterisk means HYL1–6myc. Left panel displays the morphological characteristics of WT and mutants. ( b ) The cartoon shows the details of transient gene constructs. ( c ) Transient-complementation assays. Transiently expressed COP1-YFP and DN-COP1-YFP successfully restored the level of HYL1 in cop1-6 protoplasts in contrast to COP1 Δ N-YFP, COP1 Δ C-YFP and YFP that were unsuccessful. ( d ) The expression of transfected genes were determined by confocal microscopy. ( e ) The levels of HYL1 in WT /XVE-DN-COP1-6myc and WT /XVE-COP1-6myc transgenic plants, which have grown in β-estradiol supplemented medium for 10 days. The experiments were commenced with three individual transgenic lines. The levels of HYL1 were determined with α-HYL1 antibody. Induced DN-COP1 and COP1 were determined with α-Myc antibody. Equal loading of samples was determined with α-actin antibody. Full size image To ensure the correlation between the HYL1-reduction and COP1 deficiency, we performed transient-complementation assays using cop1-6 protoplasts. Full-length COP1 , DN-COP1 (a dominant-negative COP1 with four mutations in RING-finger domain), amino (N)-terminal deletion COP1 ( COP1ΔN ) and carboxy (C)-terminal deletion COP1 ( COP1ΔC ) proteins with a yellow fluorescent protein (YFP) tag were transiently expressed in cop1-6 protoplasts ( Fig. 2b,c ). On the expression of either COP1-YFP or DN-COP1-YFP for 18 h, the level of HYL1 was dramatically increased as compared with controls ( YFP ). By contrast, neither the expression of COP1ΔC-YFP nor COP1ΔN-YFP restored the highly reduced level of HYL1 in cop1-6 protoplasts ( Fig. 2c ). The expression levels of transient genes were verified with confocal microscopy ( Fig. 2d ). The role of COP1 for the expression of HYL1 was further unravelled with transgenic plants harbouring the DN-COP1-6myc gene or the COP1-6myc gene under the control of β-estradiol inducible promoter (XVE). By increasing the concentration of β-estradiol, the inductions of DN-COP1-6myc, which represses the endogenous COP1 E3 ligase activity through dimerization [24] , or COP1-6myc in the transgenic plants were observed. The induction of either DN-COP1-6myc or COP1-6myc substantially increased the level of HYL1 in a concentration-dependent manner ( Fig. 2e ). These results suggest that COP1 maintains the expression of HYL1 independently of its ubiquitin-conjugating activity. UPS-independent post-translational proteolysis of HYL1 Even though our results have shown that COP1 is important to maintain HYL1 expression, it was unclear how COP1 modulates the level of HYL1. To elucidate whether the expression of HYL1 was modulated at the stage of mRNA or protein, we tested the levels of HYL1 and SERRATE transcripts in cop1-4 and cop1-6 by quantitative PCR with reverse transcription (QRT–PCR). SERRATE and HYL1 transcripts were not decreased by the COP1 deficiency ( Fig. 3a ). Furthermore, the RT–PCR result showed the integrity of full-length HYL1 transcript in cop1 alleles ( Fig. 3a ). Sequencing analysis also ruled out a possible nonsense mutation in HYL1 transcript that results in truncated and non-functional HYL1 translation. These results indicated that the reduction of HYL1 in cop1 is completely unrelated to the regulation of HYL1 transcripts. 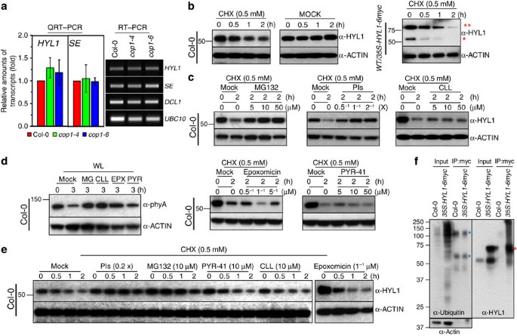Figure 3: HYL1 is a short-lived protein and highly unstable but not in ubiquitin–proteasome pathway. (a) QRT–PCR analysis ofHYL1andSERRATEtranscripts incop1-4andcop1-6. The data were collected as average value of four biological samples with ±s.d. (n=12). (b)In vivoprotein-decay assay using a translation inhibitor, cycloheximide (CHX); Left panel—wild-type seedlings with CHX, middle panel—wild-type seedlings with mock and right panel—WT/35S-HYL1-6myctransgenic seedlings with CHX. Single asterisk means endogenous HYL1; double asterisk means HYL1–6myc. (c) Concentration-dependent effects of proteolysis inhibitors on CHX-decay assay. WT seedlings were treated with CHX (0.5 mM) with or without MG132 (5, 10 and 50 μM), PIs (0.05, 0.1 and 0.2 × ), CLL (5, 10 and 50 μM), PYR-41 (5, 10 and 50 μM) or epoxomicin (0.05, 0.1 and 0.5 μM). (d) Effect of inhibitors on the stability of phyA. Seedlings were grown for 7 days under a 12-h white light/12-h darkness photoperiod and sampled 3 h after transitioning to white light. This result is an example showing the effect of UPS inhibitors on a target protein, which is regulated by ubiquitin–proteasome pathway. (e) Effects of proteolysis inhibitors on CHX-decay assay. WT seedlings were treated with CHX (0.5 mM) with or without MG132 (10 μM), PIs (0.2 × ), CLL (10 μM), PYR-41 (10 μM) or epoxomicin (0.1 μM). The levels of endogenous HYL1 were determined with α-HYL1 antibody. In all tests, the equal loading of samples was determined with α-actin antibody. (f)In vivoubiquitination analysis of co-immunoprecipitated HYL1–6myc. HYL1–6myc was precipitated with α-myc antibody and ubiquitination pattern was determined with α-Ub antibody. Blue asterisks indicate nonspecific bands. Red asterisk indicates immunoprecipitated HYL1–6myc. Figure 3: HYL1 is a short-lived protein and highly unstable but not in ubiquitin–proteasome pathway. ( a ) QRT–PCR analysis of HYL1 and SERRATE transcripts in cop1-4 and cop1-6 . The data were collected as average value of four biological samples with ±s.d. ( n =12). ( b ) In vivo protein-decay assay using a translation inhibitor, cycloheximide (CHX); Left panel—wild-type seedlings with CHX, middle panel—wild-type seedlings with mock and right panel—WT /35S-HYL1-6myc transgenic seedlings with CHX. Single asterisk means endogenous HYL1; double asterisk means HYL1–6myc. ( c ) Concentration-dependent effects of proteolysis inhibitors on CHX-decay assay. WT seedlings were treated with CHX (0.5 mM) with or without MG132 (5, 10 and 50 μM), PIs (0.05, 0.1 and 0.2 × ), CLL (5, 10 and 50 μM), PYR-41 (5, 10 and 50 μM) or epoxomicin (0.05, 0.1 and 0.5 μM). ( d ) Effect of inhibitors on the stability of phyA. Seedlings were grown for 7 days under a 12-h white light/12-h darkness photoperiod and sampled 3 h after transitioning to white light. This result is an example showing the effect of UPS inhibitors on a target protein, which is regulated by ubiquitin–proteasome pathway. ( e ) Effects of proteolysis inhibitors on CHX-decay assay. WT seedlings were treated with CHX (0.5 mM) with or without MG132 (10 μM), PIs (0.2 × ), CLL (10 μM), PYR-41 (10 μM) or epoxomicin (0.1 μM). The levels of endogenous HYL1 were determined with α-HYL1 antibody. In all tests, the equal loading of samples was determined with α-actin antibody. ( f ) In vivo ubiquitination analysis of co-immunoprecipitated HYL1–6myc. HYL1–6myc was precipitated with α-myc antibody and ubiquitination pattern was determined with α-Ub antibody. Blue asterisks indicate nonspecific bands. Red asterisk indicates immunoprecipitated HYL1–6myc. Full size image Accordingly, to test the proteolytic regulation of HYL1, we conducted protein-decay assays. Ten-day-old wild-type and WT/35S-HYL1-6myc transgenic seedlings were treated with cycloheximide (CHX) (0.5 mM) to block the de novo synthesis of HYL1. In the constrained conditions, we observed that the levels of HYL1 and HYL1–6myc dwindled during 2 h, showing that HYL1 is a relatively short-lived protein ( Fig. 3b ). Two major proteolytic pathways, the UPS and autophagy, have been defined in plants [25] , [26] . To investigate which of the two proteolytic pathways regulates the proteolysis of HYL1, we performed cycloheximide (CHX)-decay assays with or without protease inhibitor cocktail (PIs)—a blend of proteases inhibitors with a broad spectrum, Carbobenzoxy-Leu-Leu-leucinal (MG132)—a reversible proteasome inhibitor, and clasto-lactacystin β-lactone (CLL)—an irreversible proteasome inhibitor, which is more specific and has fewer side effects than MG132. As shown in Fig. 3c,e and Supplementary Fig. 4 , the additions of MG132 (5, 10, 50 μM) or PIs (0.05-, 0.1-, 0.2-fold) notably suppressed the destabilization of HYL and HYL1–6myc. In contrast, the treatments of CLL (5, 10, 50 μM) were ineffective in inhibiting HYL1 degradation. Further, we observed the ineffectiveness of epoxomicin, another irreversible proteasome inhibitor, on the blocking of HYL1 breakdown. Since UPS consists of two distinct processes, ubiquitin-conjugation and 26S proteasome-mediated proteolysis, we used PYR-41, an inhibitor for E1 enzyme by which the transfer of ubiquitin to E2 enzyme can be irreversibly retained [27] . We treated seedlings with the inhibitor (5, 10, 50 μM) to block the ubiquitin-conjugation process. The PYR-41 treatments were unable to suppress HYL1 degradation in the CHX-decay assay, indicating that the ubiquitin-conjugation process is not essential for HYL1 destabilization ( Fig. 3c,e ). To further clarify the irrelevance of ubiquitin-conjugation process for HYL1 degradation, we performed in vivo ubiquitination analysis with WT/35S-HYL1-6myc lines. Using anti-myc antibody, we co-immunoprecipated HYL1–6myc complex and determined the possible ubiquitination of HYL1–6myc with anti-Ub antibody. As shown in fig. 3f , HYL1–6myc is not ubiquitinated in vivo , confirming UPS is not responsible for HYL1 degradation. Although the investigation regarding the pathway—UPS or autophagy—into which HYL1 degrades was incoherent due to the contradictive results between MG132 and the other proteasome inhibitors, we believe that UPS is not related to the post-translational regulation of HYL1 on the basis of the results of CLL, epoxomicin and PYR-41 treatments and in vivo ubiquitination analysis. We suggest that the MG132 results may be accounted for by its strong inhibitory effects on cysteine and serine proteases (for example, calpain and cathepsins) through the formation of hemi-acetal or hemi-thioacetals with either hydroxyl or thiol nucleophiles [28] . The effects of UPS inhibitors in our experiments were verified by monitoring the stability of phytochrome A, a well-defined target protein of UPS, under continuous white light ( Fig. 3d ). HYL1 is degraded by an unknown protease X Recently, the autophagic degradation of Dicer and AGO2 was reported in animals [29] . The involvement of autophagic flux for AGO1 modulation was also found in plants [30] . In this context, we inferred the effects of PIs and MG132 on HYL1 stability as the outcome of inhibiting an autophagic protease or proteases ( Fig. 3c,e ). Prolonged treatments of several protease inhibitors such as E64D—an irreversible cysteine protease inhibitor—are known to strongly block autophagic degradation in autophagolysosome (or vacuole) [31] . Thus, we treated PIs, MG132 or E64D to 10-day-old seedlings for 18 h. Similar to the results of CHX-decaying assays ( Fig. 3 ), the long-time treatments of inhibitors dramatically increased the level of HYL1, confirming that HYL1 is degraded by a protease or proteases ( Fig. 4a–c ). At first glance, these results seemingly reflected a fact that HYL1 is degraded by autophagic proteases. However, autophagic pathway consists of multistep processes including (1) the induction of autophagopore formation, (2) the engulfing process of substrates into autophagosome and (3) the fusion of autophagosome into vacuoles/lysosomes for cargo degradation and re-use [32] . By now, it has been widely accepted that analysing a part of autophagic processes alone is an inadequate measure of autophagic degradation activity (flux). 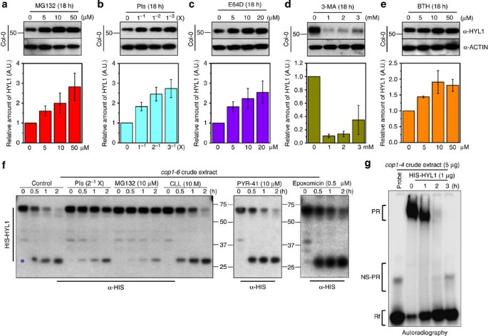Figure 4: Autophagy is not a disintegrator of HYL1. Protein blot analyses of chemically treated seedlings; (a) Seedlings were incubated with MG132 (0–50 μM). (b) Seedlings were incubated with PIs (0–3−1× ). (c) Seedlings were incubated with E64D (0–20 μM). (d) Seedlings were incubated with 3-MA (0–2 mM). (e) Seedlings were incubated with BTH (0–50 μM). The levels of HYL1 were determined with α-HYL1 antibody. Equal loading of samples was determined with α-actin antibody. The relative amounts of HYL1 were calculated by image analysis and plotted in arbitrary unit versus the level of initial sample. The data were collected as the average value of four immunoblot analyses with ±s.d. (n=4). (f)In vitrocell-free degradation assay using recombinant HYL1 andcop1-6crude extracts. PIs (0.05, 0.1, 0.2 × ) efficiently blocks the N-terminal cleavage of HYL1. Likewise, treatments of MG132 (5, 10, 50 μM) is also effective in inhibiting the N-terminal cleavage of HYL1. Addition of CLL (5, 10, 50 μM), PYR-41 (5, 10, 50 μM) or epoxomicin (0.05, 0.1 and 0.5 μM) is ineffective. The levels of recombinant HIS-HYL1 were determined with α-HIS antibody. (g) N-terminal cleavage of HYL1 abolishes the double stranded miRNA binding activity. Gel mobility shift assay was performed with32γ-ATP-labelled double-stranded RNA as a substrate for the processes HYL1 fromin vitrocell-free degradation assay. PR means Protein–RNA complex. NS-PR means nonspecific protein (originated from crude extracts)–RNA complex. Rf means free RNA substrates. Figure 4: Autophagy is not a disintegrator of HYL1. Protein blot analyses of chemically treated seedlings; ( a ) Seedlings were incubated with MG132 (0–50 μM). ( b ) Seedlings were incubated with PIs (0–3 −1 × ). ( c ) Seedlings were incubated with E64D (0–20 μM). ( d ) Seedlings were incubated with 3-MA (0–2 mM). ( e ) Seedlings were incubated with BTH (0–50 μM). The levels of HYL1 were determined with α-HYL1 antibody. Equal loading of samples was determined with α-actin antibody. The relative amounts of HYL1 were calculated by image analysis and plotted in arbitrary unit versus the level of initial sample. The data were collected as the average value of four immunoblot analyses with ±s.d. ( n =4). ( f ) In vitro cell-free degradation assay using recombinant HYL1 and cop1-6 crude extracts. PIs (0.05, 0.1, 0.2 × ) efficiently blocks the N-terminal cleavage of HYL1. Likewise, treatments of MG132 (5, 10, 50 μM) is also effective in inhibiting the N-terminal cleavage of HYL1. Addition of CLL (5, 10, 50 μM), PYR-41 (5, 10, 50 μM) or epoxomicin (0.05, 0.1 and 0.5 μM) is ineffective. The levels of recombinant HIS-HYL1 were determined with α-HIS antibody. ( g ) N-terminal cleavage of HYL1 abolishes the double stranded miRNA binding activity. Gel mobility shift assay was performed with 32 γ-ATP-labelled double-stranded RNA as a substrate for the processes HYL1 from in vitro cell-free degradation assay. PR means Protein–RNA complex. NS-PR means nonspecific protein (originated from crude extracts)–RNA complex. Rf means free RNA substrates. Full size image Hence, to clarify whether the protease or proteases are associated with the autophagy pathway, wild-type seedlings were incubated with 3-methyladenine (3-MA)—an inhibitor of type III phosphatidylinositol 3-kinases (PI3-K)—or benzothiadiazole (BTH), a salicylic acid analogue, for 18 h, to hinder or to trigger the formation of autophagosome, respectively [33] , [34] . The effects of the given chemicals on the autophagosome formation in wild-type seedlings were verified with LysoTracker Red DND-99, a cell permeable and pH-sensitive dye for staining acidic vesicular organelles (AVO) [34] . As shown in Supplementary Fig. 5 , the red fluorescence of AVO was significantly reduced by the addition of 3-MA (2 mM) as compared with control. Further, the red emissions were substantially augmented by BTH (10 μM), validating an either positive or negative effect of the chemicals on the formation of AVO ( Supplementary Fig. 5 ). 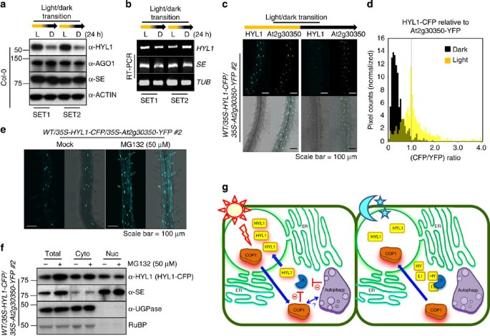Figure 5: Nucleocytoplasmic shuttling of COP1 is essential for HYL1 stability. (a) The light/dark transition assay. Ten-day-old wild-type seedlings were transferred to the continuous dark for 24 h to stimulate the nuclear remobilization of COP1. The level of HYL1 was determined with α-HYL1 antibody. AGO1 and SE were used as controls, which are not affected by the shift of COP1 into the nucleus. Equal loading of samples was determined with α-ACTIN antibody. (b) RT–PCR analysis of HYL1 and SE transcripts (c) Visualization of the dark-triggered reduction of HYL1 using WT/35S-HYL1-CFP/35S-At2g30350-YFPtransgenic seedlings. At2g30350-YFP was used as an internal control. (d) Statistical analysis of HYL1-CFP intensity versus At2g30350-YFP intensity per pixel units in the light-to-dark transition. (e) The cytoplasmic accumulation of HYL1-CFP induced by MG132. WT/35S-HYL1-CFP/35S-At2g30350-YFPtransgenic seedlings were incubated with MG132 for 18 h. The increased level of CFP fluorescence in the cytoplasmic fractions was determined by confocal microscopy. (f) Cell-fractionation-combined-immunoblot analysis. The levels of HYL1 in the nuclear fraction and cytoplasmic fraction from mock or MG132-treated double transgenic seedlings were determined with α-HYL1 antibody. SE and UGPase were used as a control for the nuclear-specific and cytoplasmic-specific fractionation, respectively. (g) A plausible model of the proteolytic regulation of HYL1 for miRNA homeostasis. On light exposure, COP1 shifts to the cytoplasm and suppresses the cleavage of HYL1 by protease X, may be, together with autophagy. In darkness, COP1 remobilizes into the nucleus that unshackles the protease X. We also observed the significant accumulations of AVO in MG132 or PIs treated seedlings and that is consistent with previous reports [31] ; PIs and MG132 enhance the accumulation of autophagosome ( Supplementary Fig 5 ). Interestingly, in contrast to our conjecture, the level of HYL1 was not efficiently retained but rather significantly diminished by 3-MA treatments ( Fig. 4d ). Under the BTH treatments, the level of HYL1 increased in relation to the enhanced intensity of red fluorescence, implying that HYL1 is not degraded by autophagy flux and the protease (or proteases) may be not functionally associated with autophagy ( Fig. 4e ). Recent studies have elucidated that UPS-coupled autophagy requires cargo adaptors and/or recognition markers (for example, ubiquitination) to mediate the case-by-substrate sequestration. The chemical blockage of UPS is known to activate the compensatory function of autophagy to remove aggregated proteins with ubiquitin tags [35] . Even though we observed that HYL1 is not subjected to ubiquitination ( Fig. 3f ), we investigated the effect of UPS inhibitors for 18 h to clearly rule out the possible involvement of UPS-coupled autophagy. In our experiments, neither the treatments of CLL nor epoxomicin altered the HYL1 levels and AVO as compared with control, implying that HYL1 is not a cargo for UPS-coupled autophagy ( Supplementary Fig. 6 ). Taken together, our results have hitherto shown that neither UPS nor autophagy is required for the immediate degradation of HYL1. Thus, we hypothesized that the degradation may be performed by an unidentified protease, provisionally named ‘X’ which falls functionally outside autophagy. To investigate the possible involvement of a non-autophagic protease, we further performed in vitro cell-free degradation assays using crude extracts from cop1 alleles (See Methods). Purified recombinant HYL1 protein with N-terminal 6 histidine-tag was incubated with cop1-4 or cop1-6 crude extract for 2 h with or without MG132, PIs, CLL, epoxomicin or PYR-41. Remarkably, HYL1 was specifically cleaved into an ~26 kDa N-terminal fragment (α-HIS antibody). While CLL, epoxomicin and PYR-41 proved to be ineffective in deterring the specific cleavage of HYL1, PIs as well as MG132 impeded the cleavage in vitro ( Fig. 4f and Supplementary Fig. 6a ). These results clearly demonstrated the highly unstable nature of HYL1 and the presence of a specific protease for HYL1 instability. Next, we investigated whether the cleavage impairs the functionality of the N terminus of HYL1 (two RNA-binding domains), which is essential for the processing of pri-miRNAs [36] , [37] . Through in vitro cell-free degradation-linked gel mobility shift assay, we found the N-terminal cleavage of HYL1 that entirely abolished the miRNA binding activity of HYL1 ( Fig. 4g ). Taken all together, these results provided two ideas; that an unidentified protease X, for the cleavage of HYL1 does not functionally belong to the autophagic pathway and moreover, that autophagy seems likely to be a positive regulator for HYL1 stability ( Supplementary Fig. 8 ). Cytoplasmic COP1 E3 ligase suppresses protease X activity COP1 harbours both nuclear import and export signal sequences, and it shuttles between the nucleus and cytoplasm in response to dark/light transition [38] , [39] . In darkness, COP1 accumulates in the nucleus, whereas upon exposure to light, COP1 rapidly migrates toward the cytoplasm. Besides, the constitutively expressed HYL1 with a fluorescence tag was mostly observed within the nucleus under light [37] ( Supplementary Fig. 9 ). Therefore, the discordance in the subcellular compartment of the two proteins raised a question wherein COP1 protects HYL1 from the protease X. To investigate the subcellular location—nucleus or cytoplasm—of the scene of defence against the proteolytic raid, we performed light-to-dark transition assays. Recent studies proposed that the remobilization kinetics of COP1 (2.4 h) from or to cytoplasm is much faster than the previously reported slow kinetics of COP1 shuttling (over 12 h), explaining the swift shuttling responses to day–night shift and even to shading [38] , [39] , [40] , [41] . Hence, wild-type seedlings were grown 10 days under continuous light (100 μmol m −2 s −1 ) and then transferred to darkness for 24 h by which the nuclear re-accumulation of COP1 could be sufficiently stimulated. As compared with the constant levels of AGO1, SE and ACTIN, a substantial reduction of HYL1 was observed, implying that cytoplasmic COP1 is important for HYL1 stability ( Fig. 5a ). In the light-to-dark transition, HYL1 transcripts were unchanged, which clearly excluded the intervention of mRNA regulatory layers ( Fig. 5b ). We also monitored the level of HYL1 in dark/light oscillations and that ensured that the stability of HYL1 is correlated to light ( Supplementary Fig. 10a ). Interestingly, the oscillation pattern of HYL1 was not observed in cop1-6 , showing that COP1 is indispensable for the light-dependent stability of HYL1 ( Supplementary Fig. 10b ). Next, the light-dependent stability was further visualized with WT/35S-HYL1-CFP/35S-At2g30350-YFP double transgenic seedlings. The fluorescence of HYL1-CFP was significantly faded from the nuclei after 24 h in darkness, unlike the relatively stable emissions from an internal control, At2g30350-YFP ( Fig. 5c ). To rule out the nonspecific decaying of HYL1-CFP, we measured the ratio of CFP versus YFP pixel by pixel in 79 (light) and 161 (dark) nuclei of two individual transgenic lines. We found that the average CFP/YFP ratio dissipated 62% in darkness from 1.24 to 0.48 ( Fig. 5d and Supplementary Fig. 9 ). Immunoblot analysis further confirmed the lowered level of HYL1-CFP in darkness ( Supplementary Fig. 10c ). Further, we treated the WT/35S-HYL1-CFP/35S-At2g30350-YFP double transgenic plants with MG132 (50 μM) for 18 h. The fluorescence of HYL1-CFP was considerably increased in cytoplasm as compared with the control ( Fig. 5e ). To further clarify the cytoplasmic accumulation, we performed the cell-fractionation combined with immunoblot assay. Consistent with the confocal analysis, the level of HYL1-CFP was mainly amassed in the cytoplasmic fraction but was unaltered in the nuclear fraction ( Fig. 5f ). The efficiency of fractionation was confirmed by the complete localization of UDP-glucose pyrophosphorylase (UGPase) in the cytoplasmic fraction and SE in the nuclear fraction. These results showed that the proteolysis of HYL1 is mostly executed in cytoplasm, possibly either before it moves into the nucleus or after it returns to the cytoplasm. Next, we added the protease inhibitors to cop1-6 seedlings to determine whether COP1 deficiency unshackles protease X, and that leads to the significant reduction of HYL1 in cop1 . The small amount of HYL1 in cop1-6 was notably amassed after 18 h treatment of PIs or MG132, implying the involvement of COP1 in curbing the protease X activity ( Supplementary Fig. 11a,b ). In other words, COP1 safeguards HYL1 from the unremitted cleavage by the protease X in cytoplasm. In conclusion, we suggest four main aspects for HYL1 destabilization; First, HYL1 may be specifically cleaved by an unidentified cytoplasmic, but non-AVO protease X. Second, COP1 E3 ligase is an indispensable element for deterring HYL1 destabilization by the protease X. Third, the nucleocytoplasmic shuttling of COP1 in response to the dark/light transition is essential in modulating HYL1 stability. Fourth, autophagy is not responsible for the degradation of HYL1 but could positively contribute to stabilize HYL1. Figure 5: Nucleocytoplasmic shuttling of COP1 is essential for HYL1 stability. ( a ) The light/dark transition assay. Ten-day-old wild-type seedlings were transferred to the continuous dark for 24 h to stimulate the nuclear remobilization of COP1. The level of HYL1 was determined with α-HYL1 antibody. AGO1 and SE were used as controls, which are not affected by the shift of COP1 into the nucleus. Equal loading of samples was determined with α-ACTIN antibody. ( b ) RT–PCR analysis of HYL1 and SE transcripts ( c ) Visualization of the dark-triggered reduction of HYL1 using WT /35S-HYL1-CFP/35S-At2g30350-YFP transgenic seedlings. At2g30350-YFP was used as an internal control. ( d ) Statistical analysis of HYL1-CFP intensity versus At2g30350-YFP intensity per pixel units in the light-to-dark transition. ( e ) The cytoplasmic accumulation of HYL1-CFP induced by MG132. WT /35S-HYL1-CFP/35S-At2g30350-YFP transgenic seedlings were incubated with MG132 for 18 h. The increased level of CFP fluorescence in the cytoplasmic fractions was determined by confocal microscopy. ( f ) Cell-fractionation-combined-immunoblot analysis. The levels of HYL1 in the nuclear fraction and cytoplasmic fraction from mock or MG132-treated double transgenic seedlings were determined with α-HYL1 antibody. SE and UGPase were used as a control for the nuclear-specific and cytoplasmic-specific fractionation, respectively. ( g ) A plausible model of the proteolytic regulation of HYL1 for miRNA homeostasis. On light exposure, COP1 shifts to the cytoplasm and suppresses the cleavage of HYL1 by protease X, may be, together with autophagy. In darkness, COP1 remobilizes into the nucleus that unshackles the protease X. Full size image Here, we presented a new perspective on the cross-talk between two extensively studied gene regulatory processes, the proteolytic decaying of proteins and miRNA-dependent mRNA clearance. In the cross-talk, COP1 plays the pivotal role as a positive console—diametrically opposite to its negative function in photomorphogenesis under visible and far-red light—in the homeostatic miRNA biogenesis in plants. Similarly, COP1 was previously reported as a positive regulator that promotes photomorphogenesis under ultraviolet-B light [42] . COP1 stabilizes long hypocotyl 5 (HY5) by forming a complex with ultraviolet-B resistance 8 (UVR8) [43] , [44] . These studies have rediscovered the function of COP1 and our finding may provide clues to understand the duplicity of COP1 in regulating protein stability. We suggested that COP1 suppresses the function of a protease X—existing but unidentified—which specifically cleaves off the N-termini of HYL1 and thereby hinders miRNA processing. Moreover, we primally showed the proteolytic regulation of HYL1 in response to the light/dark transition. The cytoplasmic partitioning of COP1 was essential in the light-dependent stabilization of HYL1. Because the RNA-binding activity of HYL1 is efficiently impaired by the proteolytic regulation, plants may be able to immediately change the levels of precisely processed miRNAs by adjusting the turnover-rate of HYL1. Even if the time-scale of regulation might be a day to several days depending on the stability of miRNAs [45] , it could be a worthwhile strategy in the instant adjustments of gene expression. For instance, we observed the COP1-dependent fluctuation of HYL1 in response to the oscillation of light/darkness ( Supplementary Fig. 10a,b ) and a recent study reported that the levels of four miRNAs (miR167, miR168, miR171 and miR398) dynamically oscillate during the diurnal cycle—accumulated by day and decreased by night—but the oscillatory pattern is not controlled by the circadian clock [46] . Therefore, the biological significance of HYL1 fluctuation can be inferred by the diurnal oscillation of short-lived miRNAs. Furthermore, Manavella et al . [12] recently reported that the function of HYL1 is regulated by CPL phosphatases. Without the activity of CPL phosphatases, HYL1 loses its functionality in accurate processing of pri-miRNAs and strand selection. In the study, it was also discussed that HYL1 hyperphosphorylation may be important for the unknown function of HYL1 in cytoplasm [12] . Considering that nucleocytoplasmic shuttling of many proteins is influenced by phosphorylation/dephosphorylation switches in eukaryotes [47] , it can be hypothesized that the hyperphosphorylated HYL1 may be transported to cytoplasm and then further destroyed under darkness. To define the link between post-translational regulation and the localization of HYL1, detailed studies have to be further implemented. We found that HYL1 is not degraded but rather stabilized by autophagy flux. Conferring HYL1 stability with the function of autophagy, the result is coherent with the recently reported finding in animals that miRNA homeostasis is modulated by autophagy, although the underlying mechanism—the degradation of DICER and AGO2—is different to our finding [29] , [45] . In animals, it was also reported that the direct association of COP1 E3 ligase and FIP200 protein—a ULK-interacting protein–is a key regulator for autophagosome formation [48] . Similarly, it is feasible to predict the presence of a cooperative interaction between COP1 and the autophagy for the homeostatic miRNA biogenesis in plants. The functional domains and biochemical properties of COP1 are highly conserved in both plants and animals. Unlike plants, animals apparently do not undergo photomorphogenesis, but animal COP1 also dynamically shuttles between nucleus and cytoplasm and the event is important for the regulation of its target proteins [49] . Therefore, our finding may provide a clue to further understand miRNA biogenesis in animals. In summary, our findings not only revealed the duplicity of COP1—a protector by day and a disintegrator by night—but also shed light on how two major regulatory pathways—light signalling and miRNA biogenesis—communicate with one another. A plausible model is shown in Fig. 5g ; during daytime, a protease X is suppressed by cytoplasmic COP1 perhaps together with autophagy through a cooperative interaction to one another. By night, COP1 shifts to the nucleus and that unshackles the activity of protease X. Accordingly, future studies on the protease X and its suppressor—COP1 and likely, autophagy—linked to light signalling pathway may open a new door to gaining knowledge of how the miRNA plasticity and homeostasis, in response to ever-changing environmental stimuli (for example, various lights; far-red, red, blue and ultraviolet) and internal signals, are dynamically regulated in plants. Hence, investigations of (1) the identification of the protease X, (2) the detailed mechanism of COP1 and autophagy underlying the suppression of the protease and (3) the integration details between light signalling and miRNA biogenesis are envisaged as next challenges. Plant materials and growth conditions Plant materials; cop1-4 , cop1-6 , XVE-DN-COP1-6myc , XVE-COP1-6myc and WT / 35S-HYL1-6myc transgenic lines were obtained from previous studies [19] , [24] , [36] . The hyl1-2, se-1, cop1-4 and cop1-6 mutants, and transgenic plants used in this study were in the Columbia background. WT / 35S-HYL1-CFP/Ag2g30350-YFP transgenic plants were introduced into plants by Agrobacterium (EHA105 strain)-mediated infiltration using the floral dip method [50] . At2g30350 encodes two putative transcripts and one of them harbours a gene for GIY-YIG domain protein, which belongs to a class of homing endonucleases. Plants were grown in three different photoperiod conditions following the purpose of experiments. For CHX-decay assay, plantlets were grown in a constant light condition (24 h, 100 μmol m −2 s −1 ). Long-day photoperiod (16 h light/8 h dark, 100 μmol m −2 s −1 ) was applied to grow WT/XVE-DN-COP1-6myc and WT/XVE-COP1-6myc plants and cop1-6 plants for the transient-complementation assay. Short-day photoperiod (12 h light/12 h dark, 100 μmol m −2 s −1 ) was applied for the phyA stabilization experiment. DNA/AgNCs-based miRNA detection DNA-GG172-12nt-RED and the DNA-12nt-RED-166 (15 μM) probes were incubated at 25 °C for 1 min in the given concentrations of Tris-acetate buffer, followed by the addition of AgNO 3 (250 μM) and NaBH 4 (250 μM), (1:17:17) to a final volume (50 μl). For the miRNA detection assay, we mixed a fixed amount of total RNAs (5 μg) from cop1-6 , hyl1-2 and wild type with the probes at the given concentrations of Tris-acetate buffer and incubated for 15 min at 25 °C. Then, AgNO 3 (250 μM) and NaBH 4 (250 μM) were added to the RNA/DNA mixtures to a final volume (50 μl) (14–17). All the DNA/AgNCs reactions were incubated for 1 h at 25 °C and diluted with 450 μl of distilled water before measurement on a fluorimeter (Horiba Jobin Yvon, Fluoromax-4) in a 10 mm disposable cuvette. RNA extraction and analyses Total RNA was extracted from Arabidopsis seedlings using RNeasy Plant Mini kits (Qiagen). Reverse transcription was performed using MMRV reverse transcriptase (Promega) according to the manufacturer’s instruction. Primers for HYL1 , SERRATE , DCL1 , TUB and UBC10 are described in Supplementary Table 1 . QRT–PCR was carried out using Rotor-Gene Q real time PCR system (Qiagen). Relative amounts of HYL1 and SERRATE transcripts were obtained by calibrating target genes’ threshold cycles with ACTIN threshold cycles. Calculations were performed using the formula 2 (−ΔΔCT) , where C T is the cycle number at which the fluorescence reached the threshold point for detection. The experiments were performed with three independent biological replicates. Small RNA isolation and northern blot analysis Total RNAs were isolated from 10-day-old seedlings using Trizol reagent (Invitrogen). The extracted aqueous phase was precipitated with 2-propanol twice (100 and 75%) and resolved in 50% formamide. Purified RNAs were resolved on 12.5–15% denaturing polyacrylamide gel (National Diagnostics) before transferring to a nylon membrane (Amersham). The 5′ end-labelled DNA probes were applied for hybridization of blots for 12 h (Ambion). Blots were washed twice with SSC (2 × )/SDS (0.1%) for 20 min each. Hybridization signals were detected with Typhoon trio phosphoimager (GE Healthcare). Deep sequencing and analysis of small RNAs Construction of small RNA libraries with Col-0, hyl1-2 and cop1 , deep sequencing and analysis of small RNAs was performed by Macrogen Ltd., Korea. The expression levels of miRNAs (transcripts per 10 million (TPTM)) in the indicated samples were calculated by normalizing miRNA counts with the total number of clean reads in the small RNA libraries. Construction of vectors for plant and bacterial expression COP1 , DN-COP1 , COP1ΔN and COP1ΔC fragments were cloned into pENTR/D, followed by LR reaction with p2GWY7 vector ( http://gateway.psb.ugent.be/ ). HIS-tag-fused HYL1 was also generated by TOPO cloning system. HYL1 full-length fragment was cloned into pENTR/D and introduced to pPROEX-DC-HTa (this study) by LR reaction. Recombinant protein expression and purification Escherichia coli , BL21 (DE3) strain, harbouring the expression vector, pPROEX-HTa-HYL1 was incubated at 37 °C for 2 h, and then incubated at 18 °C for 12 h after IPTG induction (0.4 mM). Treated cells were broken by a French pressure cell press (Constant System Ltd.) in purification buffer (20 mM Tris-Hcl at pH 7.4; 200 mM NaCl; 1 mM EDTA; 1% Triton X-100; 2 mM phenylmethylsulphonyl fluoride) containing a proteinase inhibitor cocktail (Roche). After centrifugation (20,000 r.p.m., 40 min), the supernatant was loaded onto a Ni 2+ affinity column that was equilibrated in 50 mM Tris (pH 7.6) with 500 mM NaCl. Nonspecific-binding proteins were extensively washed out by the same buffer with 25 mM imidazole, and specific-binding protein was eluted with 250 mM imidazole in the same buffer. The buffer of purified protein was exchanged with cell-free degradation buffer. Transient expression in cop1-6 protoplasts 35S-COP1-YFP , 35S-DN-COP1-YFP , 35S-COP1ΔN-YFP and 35S-COP1ΔC-YFP constructs were transformed into cop1-6 protoplasts by polyethylene glycol method [51] . To monitor the nuclear localization of COP1 and DN-COP1, after transformation, protoplasts were incubated for 18 h. under darkness. The expressions of transformed genes were monitored by confocal microscopy (CLSM Leica SP5). For the complementation assay, the transformed protoplasts were incubated under continuous light for 18 h. Transient expression experiments were performed three times with three different biological samples. cop1-6 plants were grown under long-day photoperiod. Inducible gene expression by β-estradiol treatments Ten-day-old WT/XVE-DN-COP1-6myc and WT/XVE-COP1-6myc transgenic seedlings were germinated and grown on ½ MS medium for 7 days (16 h light/8 h dark photoperiod). The seedlings were transferred to the β-estradiol supplemented ½ MS medium at the indicated concentrations and grown for 10 days. The expression levels of DN-COP1-6myc and COP1-6myc were determined by immunoblot analyses using α-myc antibody (dilution 1:4,000, Life technologies, R951-25). HYL1 and SERRATE antibodies production We generated polyclonal HYL1 and SERRATE antibodies using HIS-HYL1 and GST-SE, respectively. Specific HYL1 and SERRATE antibodies were purified from rabbit serum using protein A agarose resin. Protein gel blot analyses Ten-day-old seedlings of wild-type, hyl1-2 , se-1 and cop1 alleles were mixed with 5 × SDS sample buffer for 10 min, and extracts were resolved on 8 to 12% SDS–PAGE after boiling at 100 °C. The resolved gels were transferred to membrane. Blots were detected with α-COP1 antibody (dilution 1:500, Agrisera, AS08 342), α-DCL1 antibody (dilution 1:1,000, Agrisera, AS12 2102), α-SERRATE antibody (dilution 1:5,000, this study) and α-HYL1 antibody (dilution 1:5,000, this study). The full immunoblot image of α-HYL1 antibody was shown in Supplementary Fig. 7b . The full immunoblot image of α-SEERATE antibody was shown in Supplementary Fig. 12 . Cycloheximide (CHX)-chase assay and Chemical treatments For the CHX-chase assay, 10-day-old seedlings of wild-type and WT/35 S-HYL1-6myc transgenic plants were treated with cycloheximide (0.5 mM) or mock treatment at the indicated time (0, 0.5, 1 and 2 h) and then samples were mixed with 5 × SDS sample buffer for 10 min and the extracts were resolved on 8 to 12% SDS–PAGE after boiling at 100 °C. The seedlings were subjected to the same procedure with MG132 (Sigma), protease inhibitor cocktail tablets (PIs, Roche), E64D (Sigma), clasto-lactacystin β-lactone (CLL, Sigma), PYR-41 (Sigma) or Epoxomicin (Sigma) treatments at the indicated concentrations. Blots were detected with α-myc antibody, α-HYL1 antibody (dilution 1:5,000, this study), α-HIS-HRP antibody (dilution 1:5,000, Sigma, A7058) and α-ACTIN antibody (dilution 1:3,000, Agrisera, AS13 2640) antibodies. The relative amounts of HYL1 were calculated by image analysis programme (ImageQuantTL, GE Healthcare). For the validation of the inhibitor treatment condition, seedlings were grown for 7 days (12-h light/12-h dark photoperiod) and sampled 3 h after exposing to light with inhibitors; MG132 (10 μM), CLL (10 μM), PYR-41 (10 μM) and epoxomicin (0.5 μM). The levels of phyA were determined with α-phyA antibody (dilution 1:1,000, Agrisera, AS07 220). This result is an example showing the effect of UPS inhibitors on a target protein, which is regulated by the ubiquitin–proteasome pathway. LysoTracker staining and confocal analysis LysoTracker staining was performed according to the manufacturer’s instruction with some modification. Whole seedlings from control and chemical-treated samples were incubated with LysoTracker Red DND-99 (50 nM) for 3 h and were then washed with ½ MS medium for 2 min. All the samples were visualized under the confocal microscope, with a laser wavelength for LysoTracker (577/590 nm). To make the results comparable, laser power and channel setting were kept identical for all the samples. Light-to-dark transition assay For the light-to-dark transient assay, 10-day-old wild-type, cop1-6 and transgenic seedlings were grown under continuous light condition (100 μmol m −2 s −1 ) and transferred to darkness for 24 h. For the light/dark oscillation, plants were placed back and forth between light and dark twice. The levels of HYL1, AGO1, SE and ACTIN were determined with α-HYL1 antibody (dilution 1:5,000, this study), α-AGO1 antibody (dilution 1:3,000, Agrisera, AS09 527), α-SERRATE antibody (dilution 1:5,000, this study) and α-ACTIN antibody (dilution 1:3,000, Agrisera, AS13 2640), respectively. Confocal image analysis of HYL1-CFP/At2g30350-YFP plantlets Regions of interest (ROIs) were made in the At2g30350-YFP image using the analyse particles plugin for ImageJ [52] . A CFP/YFP ratio image was generated by dividing the HYL1-CFP image with At2g30350-YFP image, both background subtracted. Outside the ROI, pixels were set to NaN. A de-speckle function and threshold between 0 and 4 were applied before mean value of each ROI was measured and then summarized in Supplementary Table 2 . Pixel-counting histograms were made from combined light and dark CFP/YFP ratio images, respectively. Cell-fractionation assay WT/HYL1-CFP/At2g30350-YFP transgenic seedlings were homogenized in nuclear isolation buffer consisting of 20 mM Tris-HCl (pH 7.4), 25% glycerol, 20 mM KCl, 250 mM sucrose, 2.5 mM MgCl 2 , 1 mM phenylmethylsulfonyl fluoride and 1 × protease inhibitor cocktail (Roche). The extracts were filtered through the mesh and centrifuged at 1,000 g for 10 min to harvest the supernatant and pellet. The supernatant was centrifuged at 21,000 g for 30 min to harvest the cytosolic fraction and the pellet was washed twice with nuclear isolation buffer including 0.1% Triton X-100 to obtain the nuclear fraction. The efficiency of cell-fractionation assay was confirmed with two marker proteins; the level of UGPase was determined with α-UGPase antibody (dilution 1:3,000, Agrisera, AS05 086) and the level of SE was determined with α-SERRATE antibody (dilution 1:5,000, this study). In vitro cell-free degradation assay Ten-day-old seedlings of cop1-6 and cop1-4 were extracted in cell-free degradation buffer (1 × PBS, 10 mM MgCl 2 and 10% glycerol). To minimize the contamination of acid vesicular proteases, we did not add detergent to the extraction buffer. We disrupted the samples in liquid nitrogen with pestle and mortar and then purified the cytoplasmic fraction (supernatant) by high speed centrifugation (21,000 g ) for 20 min twice. Purified recombinant His-HYL1 (1 μg) was mixed with 5 μg of cop1-6 extracts and incubated at 30 °C at the indicated time (0, 0.5, 1 and 2 h) in the presence of various chemicals (MG132, PIs, clasto-lactacystin β-lactone (CLL), PYR-41 or epoxomicin. His-HYL1 was also mixed with 5 μg of cop1-4 extracts in cell-free degradation buffer and incubated with or without chemicals for 2 h at the indicated concentrations. Gel mobility shift assay Gel mobility shift assay was performed with previous protocol with minor modifications [42] . HYL1 (1 μg) was incubated with cop1-4 crude extract (5 μg) to perform in vitro cell-free degradation assay. The assay was stopped by adding PIs (0.2 × ) and then subjected for gel mobility shift assay. Duplex miR160/miR160* (2 × 10 −7 M) was labelled with 2 μl of 32 γ-ATP 6000 Ci mmol −1 (GE Healthcare) for 1 h. The labelled substrate was incubated with the in vitro cell-free degradation products with 1 unit of RNasin (Promega) for 20 min at 4 °C. Reaction mixtures were resolved on 10% non-denatured polyacrylamide gel. Results were analysed with a Typhoon trio phosphoimager (GE Healthcare) by reading autoradiography. In vivo ubiquitination analysis For in vivo detection of ubiquitinated HYL1, we used 10-day-old seedlings of wild-type and WT/ 35S-HYL1-6myc transgenic plants. Samples were ground in protein extraction buffer (1 × PBS, 10% glycerol, 10 μM MG132 and 1 × complete protease inhibitor cocktail) and were co-incubated with α-myc Affinity resin (Sigma) for 4 h. Bound proteins were eluted and ubiquitinated proteins were determined with α-ubiquitin antibody (dilution 1:10,000, Agrisera, AS08 307). Immunoprecipitated HYL1–6myc was monitored with α-HYL1 antibody (dilution 1:5,000, this study). How to cite this article : Cho, S. K. et al . COP1 E3 ligase protects HYL1 to retain microRNA biogenesis. Nat. Commun. 5:5867 doi: 10.1038/ncomms6867 (2014).